Using geospatial modelling to optimize the rollout of antiretroviral-based pre-exposure HIV interventions in Sub-Saharan Africa Antiretroviral (ARV)-based pre-exposure HIV interventions may soon be rolled out in resource-constrained Sub-Saharan African countries, but rollout plans have yet to be designed. Here we use geospatial modelling and optimization techniques to compare two rollout plans for ARV-based microbicides in South Africa: a utilitarian plan that minimizes incidence by using geographic targeting, and an egalitarian plan that maximizes geographic equity in access to interventions. We find significant geographic variation in the efficiency of interventions in reducing HIV transmission, and that efficiency increases disproportionately with increasing incidence. The utilitarian plan would result in considerable geographic inequity in access to interventions, but (by exploiting geographic variation in incidence) could prevent ~40% more infections than the egalitarian plan. Our results show that the geographic resource allocation decisions made at the beginning of a rollout, and the location where the rollout is initiated, will be crucial in determining the success of interventions in reducing HIV epidemics. Ameliorating the HIV pandemic in resource-constrained settings is one of the greatest challenges facing the global community in the 21st Century. Worldwide ~34 million individuals are infected with HIV; and in Sub-Saharan Africa alone, 3 million new infections occur annually [1] . Results from recent clinical trials indicate that prevention tools based on antiretrovirals (ARVs) could be effective in controlling the pandemic. ARV-based pre-exposure prophylaxis (PrEP) [2] , [3] , [4] , ARV-based microbicides [5] and providing ARVs to the HIV-positive partner in a discordant couple [6] have been shown to provide partial protection against HIV infection. Interventions, based on these tools, may soon be rolled out in resource-constrained countries in Sub-Saharan Africa. When this occurs, governments will have to decide how to allocate their available resources. Allocation decisions will be based on a consideration of multiple factors, including their ethical implications. The World Health Organization has recommended considering four ethical principles when deciding how to allocate scarce resources: the egalitarian principle of equity in access to the resource, the utilitarian principle of maximizing overall societal benefits, the Maximin principle (prioritizing the least advantaged individuals) and the principle of justice as reciprocity or compensation [7] , [8] . A government, operating under resource constraints, may choose to make resource allocation (RA) decisions based on one or more of these principles. Here we use geospatial modelling to compare two rollout plans: one is based on the egalitarian principle and the other on the utilitarian principle. Both plans use the same amount of resources. The objective of the egalitarian plan is to maximize countrywide equity in access to the available prevention resources. The objective of the utilitarian plan is to maximize the number of HIV infections prevented (IP). We compare the rollout plans, under resource constraints, in terms of: (i) the geographic RA strategy (GRAS) that is needed for implementation, (ii) the optimal location to begin the rollout and (iii) the number of HIV IP. In addition, we identify significant geographic variation in the efficiency of interventions in reducing HIV transmission, and a nonlinear relationship linking efficiency with the pre-intervention HIV incidence rate. We discuss the implications of our results for rolling out ARV-based microbicides, and other ARV-based pre-exposure interventions, in Sub-Saharan Africa. Women are disproportionally affected by the HIV epidemic in Sub-Saharan Africa. Therefore we chose to focus our analyses on the potential rollout of interventions using ARV-based microbicides. We evaluate rollout plans for South Africa as we use data from the landmark trial, CAPRISA 004, which was conducted in KwaZulu-Natal province in 2010 (refs 5 , 9 ). CAPRISA 004 showed that a tenofovir-based microbicide gel with coital dosing was partially effective in preventing HIV infection. The microbicide was also found to be partially effective in protecting against herpes simplex virus type 2 (HSV-2). After the success of CAPRISA 004 the South African Government began a confirmatory trial, FACTS 001, in 2011. This is a nine-site trial that uses the same microbicide and coital dosing as in CAPRISA 004. The plan is to enroll over 2,000 women; results will be available at the end of 2014. FACTS 001 is a phase III licensure study. If it is at least as successful as the CAPRISA 004 trial the microbicide could receive regulatory approval by 2015. To prepare for a potential rollout of this microbicide, the South African Government’s Technology Innovation Agency has made a licence agreement with CONRAD, the organization that supervised the manufacture of the microbicide for CAPRISA 004. This agreement grants Technology Innovation Agency the rights, if the microbicide receives regulatory approval, to manufacture and distribute the microbicide in Africa. 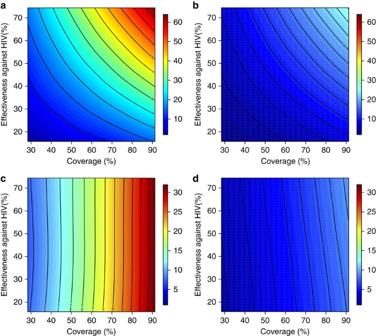Figure 1: Results of a multivariate sensitivity analysis of the geospatial meta-population transmission model Response hypersurfaces show the cumulative percentage of HIV infections prevented in KwaZulu-Natal (after 10 years of a microbicide-based intervention) as a function of the effectiveness of the microbicide against HIV and coverage for (a) women and (b) men. Response hypersurfaces show the cumulative percentage of HSV-2 infections prevented in KwaZulu-Natal (after 10 years of a microbicide-based intervention) as a function of the effectiveness of the microbicide against HIV and coverage for (c) women and (d) men. The average prevalence of HIV in South Africa is 17%, but prevalence ranges from 8% in women (6% in men) in the Western Cape to 26% in women (20% in men) in KwaZulu-Natal province, see Supplementary Table 1 for HIV prevalence levels in the remaining provinces. Owing to the significant geographic heterogeneity in prevalence we use geospatial modelling to compare the utilitarian with the egalitarian rollout plan. We linked two types of models: a geospatial RA model and a geospatial meta-population transmission (MT) model of coupled HIV and HSV-2 epidemics. Each population in the model represents the population in one of the nine provinces in South Africa, and the meta-population represents the population of the entire country. The model includes the spatial demographics of South Africa, the within-country geographic variation in HIV prevalence, the province-specific rollout of treatment (with coverage increasing from 2004 onwards, see Supplementary Fig. 1 ) and geographic heterogeneity in sexual behaviour; see Methods. Calibrating the geospatial MT model Our gender-stratified estimates of HIV incidence rates and prevalence levels, obtained from the calibration procedure (see Methods), show significant geographic variation throughout South Africa. 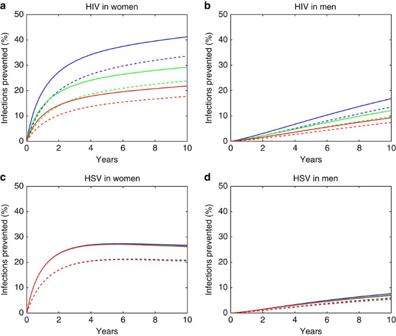Figure 2: Temporal effect of the effectiveness of the microbicide against HIV and coverage on reducing HIV and HSV-2 transmission in KwaZulu-Natal. Temporal scenarios for the cumulative percentage of HIV IP are shown for (a) women and (b) men. Temporal scenarios for the cumulative percentage of HSV-2 IP are shown for (c) women and (d) men. Blue, green and red curves depict scenarios with high, moderate and low adherence to microbicides, respectively. Note, colours overlap for (c) and (d). These adherence levels correspond to an effectiveness level in protecting against HIV infection of 54%, 38% and 28% (as in the CAPRISA 004 trial5). An effectiveness of 51% in protecting against HSV-2 infection, as found in the CAPRISA 004, is assumed for all of the scenarios. The solid and dashed curves depict scenarios where microbicide coverage is 90% and 60%, respectively. Province-specific gender-stratified estimates of HIV incidence rates, in terms of the median value and interquartile range (IQR), are given in Supplementary Table 2 . Province-specific gender-stratified estimates of both HIV and HSV-2 prevalence levels are shown in Supplementary Fig. 2 . Multivariate sensitivity analysis of the geospatial MT model The results of the multivariate sensitivity analysis of the geospatial MT model are presented as three-dimensional response hypersurfaces ( Fig. 1 ); the colours in the hypersurfaces show the percent reduction in transmission in KwaZulu-Natal, due to microbicides, over a decade. Figure 1 shows the impact of microbicides as a function of their effectiveness in protecting against HIV infection ( y axis) and the coverage of the intervention ( x axis). Figure 1a shows the reduction in HIV transmission for women, and Fig. 1b the reduction in HIV transmission for men. Figure 1c shows the reduction in HSV-2 transmission for women, and Fig. 1d the reduction in HSV-2 transmission for men. The response hypersurfaces show that, over a decade, the maximum reduction in HIV transmission in women could be as high as ~60%; however, this would only be possible if the effectiveness of the microbicide was high (~70%) and coverage reached ~90% ( Fig. 1a ). Under these conditions, HSV-2 transmission in women would be reduced by ~30% ( Fig. 1c ). Men would also benefit from microbicides, but to a lesser extent; their HIV transmission would be reduced by a maximum of 25% over a decade ( Fig. 1b ) and their HSV-2 transmission by a maximum of 10% ( Fig. 1d ). The reduction in HSV-2 transmission depends on microbicide coverage, but does not increase with an increase in effectiveness (over the range from 15 to 75%) of the microbicide against HIV ( Fig. 1c,d ). Figure 1: Results of a multivariate sensitivity analysis of the geospatial meta-population transmission model Response hypersurfaces show the cumulative percentage of HIV infections prevented in KwaZulu-Natal (after 10 years of a microbicide-based intervention) as a function of the effectiveness of the microbicide against HIV and coverage for ( a ) women and ( b ) men. Response hypersurfaces show the cumulative percentage of HSV-2 infections prevented in KwaZulu-Natal (after 10 years of a microbicide-based intervention) as a function of the effectiveness of the microbicide against HIV and coverage for ( c ) women and ( d ) men. Full size image Scenario analyses of the geospatial MT model The results from the scenario analyses show the effect of microbicide-based interventions in KwaZulu-Natal on reducing both HIV transmission ( Fig. 2a for women, Fig. 2b for men) and HSV-2 transmission ( Fig. 2c for women, Fig. 2d for men). Coverage is 90% in scenarios shown as solid lines and 60% in scenarios shown as dotted lines. Red, green and blue lines represent scenarios where adherence is low (red), moderate (green) or high (blue); the corresponding effectiveness of the microbicide against HIV infection is 28%, 38% and 54%. In all scenarios, regardless of adherence, the effectiveness of the microbicide against HSV-2 infection is 51%. See Methods for the definitions of adherence and effectiveness, and their relation to data from the CAPRISA 004 trial. Figure 2: Temporal effect of the effectiveness of the microbicide against HIV and coverage on reducing HIV and HSV-2 transmission in KwaZulu-Natal. Temporal scenarios for the cumulative percentage of HIV IP are shown for ( a ) women and ( b ) men. Temporal scenarios for the cumulative percentage of HSV-2 IP are shown for ( c ) women and ( d ) men. Blue, green and red curves depict scenarios with high, moderate and low adherence to microbicides, respectively. Note, colours overlap for ( c ) and ( d ). These adherence levels correspond to an effectiveness level in protecting against HIV infection of 54%, 38% and 28% (as in the CAPRISA 004 trial [5] ). An effectiveness of 51% in protecting against HSV-2 infection, as found in the CAPRISA 004, is assumed for all of the scenarios. The solid and dashed curves depict scenarios where microbicide coverage is 90% and 60%, respectively. Full size image The percentage of HIV IP in women increases quickly for ~3 years; it then continues to increase but at a slower rate ( Fig. 2a ). The greater the effectiveness of the microbicide against HIV and/or the higher the coverage the more HIV infections are prevented ( Fig. 2a ). The percentage of HIV IP in men continues to steadily increase over a decade, but is always significantly lower than in women ( Fig. 2b ). Reduction in HIV transmission in men is a delayed effect because of the indirect benefit of microbicides. The percent reduction in HSV-2 transmission in women increases quickly for 2–3 years, but then plateaus ( Fig. 2c ). The higher the coverage, the more HSV-2 IP; however, the degree of effectiveness against HIV (over the range: ~15 to ~75%) has virtually no effect on the number of HSV-2 IP ( Fig. 2c,d ). The percentage of HSV-2 IP in men continues to steadily increase over a decade, but is always significantly lower than in women ( Fig. 2d ). The effect of the HSV-2 epidemic on increasing HIV transmission in South Africa is due to the high prevalence of HSV-2 (~60% in women and ~40% in men), and a reduction in HSV-2 transmission would not lead to a reduction in HSV-2 prevalence for several decades. Consequently, the additional ‘benefit’ of the CAPRISA microbicide (that is, the effect of the microbicide in partially protecting against HSV-2 infection) will not substantially increase its impact on reducing HIV transmission over the time period of our analyses (that is, over a decade). Predictive maps of the cumulative number of HIV IP The cumulative number of HIV IP in each province, over a decade, is shown in Fig. 3 ; the predictions are based on assuming a high coverage (~90%) of the intervention. Predictions that are based on assuming moderate coverage (~60%) are shown in Supplementary Fig. 3 . The predictive maps in Fig. 3 and Supplementary Fig. 3 show median values calculated from uncertainty analyses; see Methods. 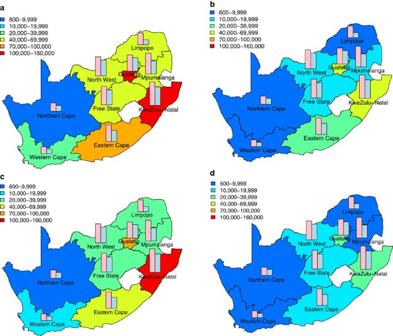Figure 3: Prediction maps of the number of HIV infections prevented (IP) in South Africa after a decade of microbicide-based interventions. The white area (within the country) represents the Kingdom of Lesotho. Pink and blue bars indicate the HIV prevalence in women and men, respectively, in each province at the beginning of the intervention. The maps show the median values of the number of HIV IP in women (a,c) and men (b,d). The estimates are based on the results of uncertainty analyses of the geospatial meta-population transmission model; in these analyses microbicide coverage reaches ~90%. To generate (a) and (b) it was assumed the effectiveness of the microbicide in protecting against HIV infection was high (median value: 54%), to generate (c) and (d) it was assumed the effectiveness of the microbicide was moderate (median value: 38%); the adherence–effectiveness relationship is based on data from the CAPRISA 004 trial5. In (a–d), the effectiveness of the microbicide in protecting against HSV-2 infection is 51% (median value)5. Figure 3a for women and Fig. 3b for men are based on assuming a high level of adherence. Figure 3c for women and Fig. 3d for men are based on assuming a moderate level of adherence. Both coverage and adherence determine the absolute number of HIV IP ( Fig. 3 ; Supplementary Fig. 3 ): the greater the coverage and/or the higher the adherence the more HIV IP. The histograms in the prediction maps show the gender-stratified prevalence of HIV in each province at the beginning of the rollout: prevalence in women (pink) and in men (blue). For comparison, histograms are scaled to the same degree in each province: province-specific prevalence levels are given in Supplementary Table 1 . Figure 3: Prediction maps of the number of HIV infections prevented (IP) in South Africa after a decade of microbicide-based interventions. The white area (within the country) represents the Kingdom of Lesotho. Pink and blue bars indicate the HIV prevalence in women and men, respectively, in each province at the beginning of the intervention. The maps show the median values of the number of HIV IP in women ( a , c ) and men ( b , d ). The estimates are based on the results of uncertainty analyses of the geospatial meta-population transmission model; in these analyses microbicide coverage reaches ~90%. To generate ( a ) and ( b ) it was assumed the effectiveness of the microbicide in protecting against HIV infection was high (median value: 54%), to generate ( c ) and ( d ) it was assumed the effectiveness of the microbicide was moderate (median value: 38%); the adherence–effectiveness relationship is based on data from the CAPRISA 004 trial [5] . In ( a – d ), the effectiveness of the microbicide in protecting against HSV-2 infection is 51% (median value) [5] . Full size image Aggregating the results over all nine provinces, we predict that the total number of HIV IP over a decade in South Africa due to microbicide-based interventions would be: 580,000 (median: IQR 500,000–670,000) in women and 190,000 (median: IQR 160,000–230,000) in men if adherence and coverage are high; 410,000 (median: IQR 340,000–490,000) in women and 136,000 (median: IQR 110,000–170,000) in men if adherence is moderate and coverage is high; 360,000 (median: IQR 310,000–420,000) in women and 110,000 (median: IQR 93,000–140,000) in men if adherence is high and coverage is moderate; 260,000 (median: IQR 210,000–300,000) in women and 81,000 (median: IQR 65,000–100,000) in men if both adherence and coverage are moderate. Intervention efficiency maps The long-term efficiency of interventions in reducing HIV transmission shows substantial geographic variation throughout South Africa ( Fig. 4 , which is based on assuming coverage is high (~90%)). Long-term efficiency is defined in terms of the number of women-years on microbicides that are needed to prevent one HIV infection in women or one HIV infection in men; efficiency increases as the number of women-years needed to prevent one HIV infection decreases. The intervention efficiency maps in Fig. 4 show median values calculated from uncertainty analyses of the geospatial MT model; see Methods. 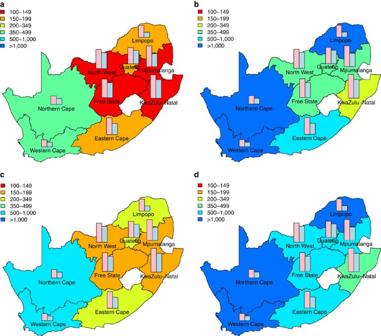Figure 4: Intervention efficiency maps for microbicide-based interventions in South Africa. The white area (within the country) represents the Kingdom of Lesotho. Pink and blue bars indicate the HIV prevalence in women and men, respectively, in each province at the beginning of the intervention. The maps show the median values of the number of women-years on microbicides that would be necessary to prevent one HIV infection in women (a,c) or men (b,d). The estimates are based on the results of uncertainty analyses of the geospatial meta-population transmission model; in these analyses microbicide coverage reaches ~90%. To generate (a) and (b) it was assumed the effectiveness of the microbicide in protecting against HIV infection was high (median value: 54%), to generate (c) and (d) it was assumed the effectiveness of the microbicide was moderate (median value: 38%); the adherence–effectiveness relationship is based on data from the CAPRISA 004 trial5. In (a–d), the effectiveness of the microbicide in protecting against HSV-2 infection is 51% (median value)5. Figure 4a,b are based on high adherence, Fig. 4c,d on moderate adherence; Fig. 4a,c show intervention efficiency maps for women, Fig. 4b,d for men. The maps show that the gender-specific intervention will reduce HIV transmission in men, as well as in women; although, not surprisingly microbicide-based interventions will be less efficient in reducing HIV transmission in men than in women. For example, in KwaZulu-Natal ~3 times more women-years are needed to prevent one HIV infection in men than to prevent one HIV infection in women. The intervention efficiency maps in Fig. 4 (based on the colour-coding) show that the nine provinces can be classified into three groups based on the long-term efficiency of interventions in reducing HIV transmission in women: high long-term efficiency (KwaZulu-Natal, Mpumalanga, the Free State and the North West Province), moderate long-term efficiency (Guateng, Limpopo and the Eastern Cape) and low long-term efficiency (the Northern and Western Cape). Results are similar for men. The difference in long-term efficiency among the provinces is substantial; for example, in KwaZulu-Natal only ~110 women-years (median value) are needed to prevent one HIV infection in women, whereas ~450 women-years (median value) are needed in the Western Cape ( Fig. 4a ). Figure 4: Intervention efficiency maps for microbicide-based interventions in South Africa. The white area (within the country) represents the Kingdom of Lesotho. Pink and blue bars indicate the HIV prevalence in women and men, respectively, in each province at the beginning of the intervention. The maps show the median values of the number of women-years on microbicides that would be necessary to prevent one HIV infection in women ( a , c ) or men ( b , d ). The estimates are based on the results of uncertainty analyses of the geospatial meta-population transmission model; in these analyses microbicide coverage reaches ~90%. To generate ( a ) and ( b ) it was assumed the effectiveness of the microbicide in protecting against HIV infection was high (median value: 54%), to generate ( c ) and ( d ) it was assumed the effectiveness of the microbicide was moderate (median value: 38%); the adherence–effectiveness relationship is based on data from the CAPRISA 004 trial [5] . In ( a – d ), the effectiveness of the microbicide in protecting against HSV-2 infection is 51% (median value) [5] . Full size image The long-term efficiency of interventions in reducing HIV transmission decreases with adherence, Fig. 4 . Notably, coverage (over the range 60–90%) has essentially no effect on the long-term efficiency of interventions; results shown in Fig. 4 are for high coverage (~90%) and those shown in Supplementary Fig. 4 are for moderate coverage (~60%). The pre-intervention incidence rate determines efficiency We found that the pre-intervention HIV incidence rate determines the long-term efficiency of interventions in reducing HIV transmission in both women ( Fig. 5 ) and men ( Fig. 6 ): the higher the HIV incidence rate, the greater the long-term efficiency. Also the higher the adherence, the greater the efficiency: Figs 5a and 6a are based on high adherence, Figs 5b and 6b on moderate adherence. The long-term efficiency of interventions in reducing HIV transmission in men is substantially lower than in women, as shown by the difference in scale on the y axis between Figs 5 and 6 . The colour code for each of the nine provinces is given in the figure legends. Data clouds are shown as these results are generated from uncertainty analyses of the geospatial MT model; see Methods. Notably, the relationship between the pre-intervention HIV incidence rate and the long-term efficiency of interventions in preventing HIV infection in both genders is highly nonlinear: efficiency increases disproportionately with increasing incidence rates. Results in Fig. 5c show the relationship between the incidence rate and the long-term efficiency of interventions when the pre-intervention HIV incidence rate is moderate to high (3–10%); again the higher the adherence, the greater the efficiency (the solid red line represents high adherence, the dotted red line moderate adherence). If adherence is high the relationship between the number of women-years needed to prevent one HIV infection, y , in women and the average pre-intervention incidence rate in women, x , can be specified by y= 1/0.00499 x ; see Methods. If adherence is moderate the relationship can be specified by y= 1/0.00361 x . 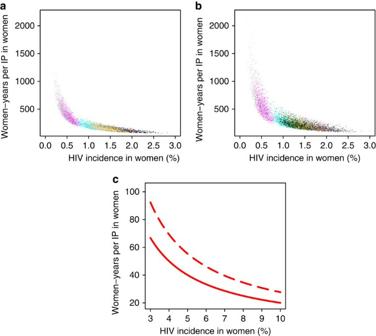Figure 5: Estimates of the province-specific long-term (that is, over a decade) efficiency of microbicide-based interventions in reducing HIV transmission in women. Long-term efficiency is shown in terms of the number of women-years on microbicides that would be necessary to prevent one HIV infection in women. Long-term efficiency increases as the number of women-years needed to prevent one HIV infection decreases. Estimates are based on the results of an uncertainty analysis of the geospatial meta-population transmission model. (a) Results are based on assuming high adherence (where high adherence is defined as in the CAPRISA trial5,9; that is, microbicides are used in >80% of sex acts). (b) Results are based on assuming moderate adherence (where moderate adherence is defined as in the CAPRISA trial5,9; that is, microbicide are used in 50–80% of sex acts). Colour codes shown inaandbrepresent: Mpumalanga (blue), Eastern Cape (green), KwaZulu-Natal (black), Limpopo (cyan), Free State (red), North West (yellow), Northern Cape (magenta), Gauteng (pink) and the Western Cape (grey). (c) Estimated number of women-years on microbicides that would be necessary to prevent one HIV infection in women living in areas where incidence in women is moderate to high when the rollout begins, assuming either high adherence (solid red line) or moderate adherence (dotted red line). Figure 5c shows, that under certain conditions, the long-term efficiency of interventions could be extremely high. For example, if interventions are rolled out in areas where HIV incidence rates in women are high (for example, 10%) and adherence is high, only ~20 women-years on microbicides would be needed to prevent one HIV infection in women ( Fig. 5c ). Figure 5: Estimates of the province-specific long-term (that is, over a decade) efficiency of microbicide-based interventions in reducing HIV transmission in women. Long-term efficiency is shown in terms of the number of women-years on microbicides that would be necessary to prevent one HIV infection in women. Long-term efficiency increases as the number of women-years needed to prevent one HIV infection decreases. Estimates are based on the results of an uncertainty analysis of the geospatial meta-population transmission model. ( a ) Results are based on assuming high adherence (where high adherence is defined as in the CAPRISA trial [5] , [9] ; that is, microbicides are used in >80% of sex acts). ( b ) Results are based on assuming moderate adherence (where moderate adherence is defined as in the CAPRISA trial [5] , [9] ; that is, microbicide are used in 50–80% of sex acts). Colour codes shown in a and b represent: Mpumalanga (blue), Eastern Cape (green), KwaZulu-Natal (black), Limpopo (cyan), Free State (red), North West (yellow), Northern Cape (magenta), Gauteng (pink) and the Western Cape (grey). ( c ) Estimated number of women-years on microbicides that would be necessary to prevent one HIV infection in women living in areas where incidence in women is moderate to high when the rollout begins, assuming either high adherence (solid red line) or moderate adherence (dotted red line). 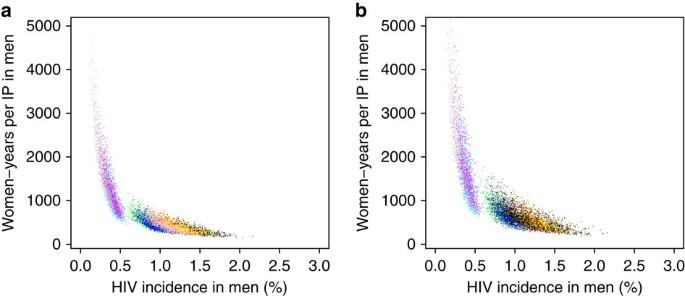Figure 6: Estimates of the province-specific long-term (that is, over a decade) efficiency of microbicide-based interventions in reducing HIV transmission in men. Long-term efficiency is shown in terms of the number of women-years on microbicides that would be necessary to prevent one HIV infection in men. Long-term efficiency increases as the number of women-years needed to prevent one HIV infection decreases. Estimates are based on the results of an uncertainty analysis of the geospatial meta-population transmission model. (a) Results are based on assuming high adherence (where high adherence is defined as in the CAPRISA trial5,9; that is, microbicides are used in >80% of sex acts). (b) Results are based on assuming moderate adherence (where moderate adherence is defined as in the CAPRISA trial5,9; that is, microbicide are used in 50−80% of sex acts). Colour codes shown inaandbrepresent: Mpumalanga (blue), Eastern Cape (geen), KwaZulu-Natal (black), Limpopo (cyan), Free State (red), North West (yellow), Northern Cape (magenta), Gauteng (pink) and the Western Cape (grey). Full size image Figure 6: Estimates of the province-specific long-term (that is, over a decade) efficiency of microbicide-based interventions in reducing HIV transmission in men. Long-term efficiency is shown in terms of the number of women-years on microbicides that would be necessary to prevent one HIV infection in men. Long-term efficiency increases as the number of women-years needed to prevent one HIV infection decreases. Estimates are based on the results of an uncertainty analysis of the geospatial meta-population transmission model. ( a ) Results are based on assuming high adherence (where high adherence is defined as in the CAPRISA trial [5] , [9] ; that is, microbicides are used in >80% of sex acts). ( b ) Results are based on assuming moderate adherence (where moderate adherence is defined as in the CAPRISA trial [5] , [9] ; that is, microbicide are used in 50−80% of sex acts). Colour codes shown in a and b represent: Mpumalanga (blue), Eastern Cape (geen), KwaZulu-Natal (black), Limpopo (cyan), Free State (red), North West (yellow), Northern Cape (magenta), Gauteng (pink) and the Western Cape (grey). Full size image Estimating the short-term efficiency of interventions The short-term (that is, in the first year of a rollout) efficiency of interventions in reducing HIV transmission, as does the long-term efficiency ( Fig. 4 ), shows substantial geographic variation throughout South Africa ( Fig. 7a,b ); short-term efficiency is defined in terms of the number of HIV IP per 10,000 microbicides in the first year of a rollout. The boxplots in Fig. 7a,b show the estimates for the short-term efficiency of interventions in reducing HIV incidence rates in women in each province. These results were calculated based on uncertainty analyses of the geospatial MT model; see Methods. The variation in the estimates of short-term efficiency, shown in the boxplots, is due to the uncertainty in the estimates of the province-specific pre-intervention HIV incidence rate in women and in the province-specific estimates of the average number of new sex partners per woman per year (see Supplementary Tables 2 and 3 ). Adherence has only a minor effect on short-term efficiency: Fig. 7a is based on high adherence, Fig. 7b on moderate adherence. Short-term efficiency, assuming high adherence, ranges from a high of 2.55 (median: IQR 2.31–2.81) HIV IP in women per 10,000 microbicides in Mpumalanga to a low of 0.81 (median: IQR 0.69–0.92) HIV IP in women per 10,000 microbicides in the Western Cape ( Fig. 7a ). Notably, Mpumalanga and KwaZulu-Natal appear to be the provinces where the short-term efficiency of interventions would be the highest, and the Northern and Western Cape the provinces where the short-term efficiency would be the lowest. However, because there is considerable overlap in the within-province estimates of efficiency, the results shown in Fig. 7a,b cannot be used to identify the province where interventions would be the most efficient in the first year of a rollout or to determine a priority ranking of provinces based on short-term efficiency. 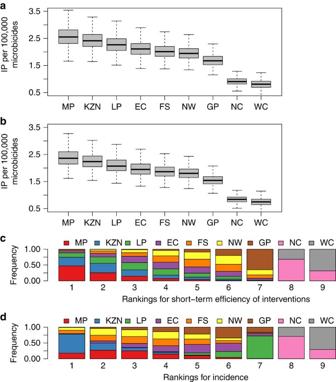Figure 7: Estimated short-term efficiency of microbicide-based interventions in reducing HIV transmission and priority rankings for provinces provinces. The boxplots inaandbshow the estimated number of HIV infections prevented in women per 10,000 microbicides in each of the nine provinces in the first year of a rollout (that is, short-term efficiency); (a) is based on high adherence, (b) on moderate adherence. The results for (a) and (b) were obtained from an uncertainty analysis of the geospatial meta-population transmission model. Province abbreviations in (a) and (b): Mpumalanga (MP), KwaZulu-Natal (KZN), Limpopo (LP), Eastern Cape (EC), Free State (FS), North West (NW), Gauteng (GP), Northern Cape (NC) and the Western Cape (WC). The black lines represent median values; the grey rectangles delimit the interquartile range. The stacked histograms incshow the probability of the priority ranking for provinces based on a probabilistic analysis of the short-term efficiency estimates shown in (a). The stacked histograms in (d) show the probability of the priority ranking for provinces based on a probabilistic analysis of the estimated pre-intervention HIV incidence rates estimated from the geospatial meta-population transmission model. Colour codes in (c) and (d) represent: Mpumalanga (red), Eastern Cape (purple), KwaZulu-Natal (blue), Limpopo (green), Free State (orange), North West (yellow), Northern Cape (pink), Gauteng (brown) and the Western Cape (grey). Figure 7: Estimated short-term efficiency of microbicide-based interventions in reducing HIV transmission and priority rankings for provinces provinces. The boxplots in a and b show the estimated number of HIV infections prevented in women per 10,000 microbicides in each of the nine provinces in the first year of a rollout (that is, short-term efficiency); ( a ) is based on high adherence, ( b ) on moderate adherence. The results for ( a ) and ( b ) were obtained from an uncertainty analysis of the geospatial meta-population transmission model. Province abbreviations in ( a ) and ( b ): Mpumalanga (MP), KwaZulu-Natal (KZN), Limpopo (LP), Eastern Cape (EC), Free State (FS), North West (NW), Gauteng (GP), Northern Cape (NC) and the Western Cape (WC). The black lines represent median values; the grey rectangles delimit the interquartile range. The stacked histograms in c show the probability of the priority ranking for provinces based on a probabilistic analysis of the short-term efficiency estimates shown in ( a ). The stacked histograms in ( d ) show the probability of the priority ranking for provinces based on a probabilistic analysis of the estimated pre-intervention HIV incidence rates estimated from the geospatial meta-population transmission model. Colour codes in ( c ) and ( d ) represent: Mpumalanga (red), Eastern Cape (purple), KwaZulu-Natal (blue), Limpopo (green), Free State (orange), North West (yellow), Northern Cape (pink), Gauteng (brown) and the Western Cape (grey). Full size image Ranking provinces based on the efficiency of interventions We used a probabilistic analysis to identify the provinces where interventions are most likely to have the highest efficiency in reducing HIV incidence in women in the first year of a rollout. To conduct this analysis, we stochastically reordered the estimates of short-term efficiency, independently for each province. Results are shown in Fig. 7c in the form of stacked histograms: rank 1 indicates the province where interventions would be the most efficient and rank 9 the province where they would be the least efficient. These results show that it is most probable that interventions would be the most efficient in two provinces (KwaZulu-Natal and Mpumalanga), but it cannot be determined whether they would be the most efficient in KwaZulu-Natal or in Mpumalanga. Furthermore, it is highly probable that the Northern and the Western Cape are the provinces where interventions are most likely to be the least efficient in the first year of a rollout ( Fig. 7c ). The North West province is likely to be in the 6th place and Guateng in the 7th place, but the rank ordering of Limpopo, the Eastern Cape and the Free State in terms of the 3rd, 4th and 5th places is not clear ( Fig. 7c ). Notably, the probabilistic ranking based on short-term efficiency estimates ( Fig. 7c ) is not exactly the same as a probabilistic ranking based on long-term efficiency estimates. This is because over time (in our case, a decade) HIV incidence rates will decrease (for both genders), as a function of increased coverage of treatment and the effects of the intervention, and the long-term efficiency of interventions is a nonlinear function of the HIV incidence rate ( Figs 5 and 6 ). Ranking provinces based on HIV incidence rates We also used a probabilistic analysis to determine the geographic regions where HIV incidence rates in women are currently the highest; to conduct this analysis we stochastically reordered the estimates for HIV incidence rates, independently for each province. These results are shown in Fig. 7d , where rank 1 indicates the province with the highest HIV incidence in women and rank 9 the province with the lowest HIV incidence. These results show that it cannot be concluded with certainty which province has the highest HIV incidence rate, but that it is most probably KwaZulu-Natal. Clearly, the Northern Cape and the Western Cape are provinces where HIV incidence is most likely to be the lowest ( Fig. 7d ). The ranking of the provinces based on estimates of HIV incidence rates is similar to the ranking based on estimates of the long-term efficiency of interventions. However, the ranking of the provinces based on estimates of HIV incidence rates ( Fig. 7d ) is not exactly the same as the ranking of the provinces based on estimates of short-term efficiency ( Fig. 7c ). This is because short-term efficiency depends upon both HIV incidence and the levels of sexual behaviour (see Methods). For example, if two provinces have the same HIV incidence rate but women in province A have (on average) slightly more partners than women in province B, interventions would be more efficient in reducing HIV transmission in province B than in province A. If the number of sex partners were exactly the same in every province (and incidence rates were known with certainty) then a ranking of the provinces based on short-term efficiency would be the same as a ranking based on HIV incidence rates. The GRAS for implementation of the utilitarian rollout plan The GRAS for implementing the utilitarian rollout plan, under different levels of resource constraints, is shown by the pie charts in Fig. 8a,b ; in both charts it is assumed that adherence is high. These results were obtained from a single optimization analysis where it was assumed that there was no uncertainty in estimating province-specific pre-intervention HIV incidence rates in women, province-specific pre-intervention HIV prevalence levels in women or province-specific levels of risk behaviour (see Methods); the objective of the optimization was to maximize the number of HIV IP throughout South Africa. Results in Fig. 8a are based on assuming there are 50 million microbicides to allocate in the first year of the rollout, this is enough for 35% of the 15–49-year-old HIV-negative women in South Africa. Results in Fig. 8b are based on assuming there are 100 million microbicides to allocate, this is enough for 65% of the 15–49-year-old HIV-negative women in South Africa. The optimization results show that under the utilitarian plan interventions should only be allocated to two of the nine provinces: Mpumalanga and KwaZulu-Natal ( Fig. 8a,b ). Therefore the optimal geographic location to rollout the utilitarian plan is in these two provinces. Mpumalanga and KwaZulu-Natal are the provinces where it is most probable that interventions would be the most efficient in reducing HIV incidence in women ( Fig. 7c ), and where HIV incidence in women is likely to be the highest ( Fig. 7d ). Similar results are obtained if adherence is moderate ( Supplementary Fig. 5 ). 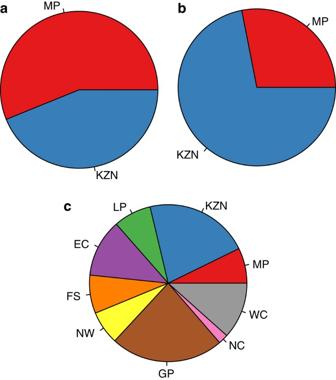Figure 8: The geographic resource allocation strategy (GRAS) for three rollout plans. The GRAS is shown (in the form of a pie chart) in terms of the proportion of the supply of microbicides that need to be allocated to each province in the first year of the rollout; all three plans are based on high adherence. The chart in (a) shows the GRAS that is necessary for the implementation of a utilitarian plan if 50 million microbicides are available (enough for ~33% of the 15–49-year-old HIV-negative women in South Africa). The chart in (b) shows the GRAS that is necessary for the implementation of a utilitarian plan if 100 million microbicides are available (enough for ~66% of the 15–49-year-old HIV-negative women in South Africa). The chart in (c) shows the GRAS that is necessary to implement the egalitarian rollout plan; it is the same whether 50 or 100 million microbicides are available. For (a–c), the province abbreviations are: Mpumalanga (MP), KwaZulu-Natal (KZN), Limpopo (LP), Eastern Cape (EC), Free State (FS), North West (NW), Gauteng (GP), Northern Cape (NC) and the Western Cape (WC). Figure 8: The geographic resource allocation strategy (GRAS) for three rollout plans. The GRAS is shown (in the form of a pie chart) in terms of the proportion of the supply of microbicides that need to be allocated to each province in the first year of the rollout; all three plans are based on high adherence. The chart in ( a ) shows the GRAS that is necessary for the implementation of a utilitarian plan if 50 million microbicides are available (enough for ~33% of the 15–49-year-old HIV-negative women in South Africa). The chart in ( b ) shows the GRAS that is necessary for the implementation of a utilitarian plan if 100 million microbicides are available (enough for ~66% of the 15–49-year-old HIV-negative women in South Africa). The chart in ( c ) shows the GRAS that is necessary to implement the egalitarian rollout plan; it is the same whether 50 or 100 million microbicides are available. For ( a – c ), the province abbreviations are: Mpumalanga (MP), KwaZulu-Natal (KZN), Limpopo (LP), Eastern Cape (EC), Free State (FS), North West (NW), Gauteng (GP), Northern Cape (NC) and the Western Cape (WC). Full size image The GRAS for implementing the utilitarian rollout plan, given 50 million microbicides, is to give 56% to Mpumalanga and 44% of the supply to KwaZulu-Natal ( Fig. 8a ). The GRAS for implementing the utilitarian rollout plan, given 100 million microbicides, is to give 72% of the supply to KwaZulu-Natal and 28% to Mpumalanga ( Fig. 8b ). When only 50 million microbicides are available there are not enough microbicides to give them to all the HIV-negative women who want them in both Mpumalanga and KwaZulu-Natal. Because it is slightly more probable that interventions will be more efficient in the first year of a rollout in Mpumalanga than KwaZulu-Natal ( Fig. 7c ), the optimization algorithm first allocates the available resources to Mpumalanga to provide microbicides to all the women who want them and then allocates the remaining resources to KwaZulu-Natal. Consequently, under this level of resource constraint Mpumalanga receives slightly more of the available resources than KwaZulu-Natal. However, when 100 million microbicides are available, Mpumalanga still receives the same number of microbicides (that is, enough to provide to all the women who want them), but there are now many more leftover to give to KwaZulu-Natal. Consequently, under this level of resource constraint, KwaZulu-Natal receives more of the available resources than Mpumalanga. The GRAS for implementation of the egalitarian rollout plan The egalitarian plan is implemented by using a proportional GRAS; this is the conventional approach for sharing a limited supply of resources, and it results in the same coverage level in every province. Using the proportional GRAS, the proportion of the supply given to each province is equal to the number of HIV-negative women living in that province divided by the total number of HIV-negative women in South Africa. This GRAS is shown by the pie chart in Fig. 8c that shows that the resources should be shared among all nine provinces. The percentage of the supply of microbicides that should be given to each province ranges from 2% (for the Northern Cape) to 21% (for Guateng province). These results show that interventions should be rolled out, simultaneously, in all nine provinces. Notably, the GRAS for the egalitarian plan only depends upon the geographic distribution of the population of HIV-negative women in South Africa; it does not depend upon the level of resource constraints. If there were no resource constraints, the GRAS for implementing the utilitarian rollout plan would be the same as the GRAS for the egalitarian plan. Number of HIV IP under the utilitarian or egalitarian plan If 50 million microbicides are available and adherence is high, using the GRAS for the utilitarian plan (shown in Fig. 8a ) would prevent 41% more HIV infections in South Africa in the first year of the rollout than the egalitarian plan: ~14,100 HIV IP versus ~10,000 HIV IP. If the same number of microbicides are available and adherence is moderate, using the GRAS for the utilitarian plan (shown in Supplementary Fig. 5a ) would prevent ~40% more HIV infections in South Africa in the first year of the rollout than the egalitarian plan: ~12,800 HIV IP versus ~9,200 HIV IP. If 100 million microbicides are available and adherence is high, using the GRAS for the utilitarian plan (shown in Fig. 8b ) would prevent ~38% more HIV infections in South Africa in the first year of the rollout than the egalitarian plan: ~27,500 HIV IP versus ~20,000 HIV IP. If the same number of microbicides are available and adherence is moderate, using the GRAS for the utilitarian plan (shown in Supplementary Fig. 5b ) would prevent ~34% more HIV infections in South Africa in the first year of the rollout than the egalitarian plan: ~24,600 HIV IP versus ~18,400 HIV IP. Including uncertainty when designing rollout plans Results from multiple (1,362 were conducted, see Methods) optimization analyses that include uncertainty in the province-specific estimates of the pre-intervention HIV incidence rates in women, the pre-intervention HIV prevalence levels in women and the levels of risk behaviour are shown in Table 1 . In these analyses the rank ordering of the provinces, in terms of HIV incidence rates in women, was varied probabilistically. Each optimization analysis calculated the GRAS necessary for implementing the utilitarian plan, and identified the optimal location for initiating the rollout in terms of a combination of two provinces. It was assumed that 50 million microbicides would be available. The combinations that occurred most frequently from the multiple optimization analyses are shown in Table 1 . The most frequent combination was Mpumalanga and KwaZulu-Natal—the same two provinces that were identified in the initial optimization analysis that did not include uncertainty. However, this specific combination was only found in 37% of the optimizations; this occurred because it is not certain in which of several provinces interventions would be the most efficient in reducing HIV incidence in women ( Fig. 7c ). Our results show it cannot be concluded with certainty that Mpumalanga and KwaZulu-Natal are the optimal combination of provinces to begin the rollout, but it should be noted that this combination occurred twice as frequently as the next most frequent two-province combination ( Table 1 ). Table 1 The results from multiple (1,362) optimization analyses that include parameter estimation uncertainty. Full size table In all of the optimization analyses, rolling out interventions using the utilitarian plan prevented substantially more HIV infections in women in the first year of the rollout than using the egalitarian plan. However, due to the uncertainty in parameter estimation, the results show fairly wide variation in terms of the allocation of resources between Mpumalanga and KwaZulu-Natal (that is, in the GRAS necessary for implementing the utilitarian plan), Table 1 . Even when Mpumalanga and KwaZulu-Natal are identified as the optimal two provinces to begin the rollout there is fairly wide variation in the GRAS. This is because in ~50% of the optimizations Mpumalanga was identified as the province where interventions would be the most efficient in the first year of the rollout in reducing HIV incidence rates in women ( Fig. 7c ) and was therefore allocated the largest proportion of resources, and in ~50% KwaZulu-Natal was identified as the province where short-term efficiency would be the highest ( Fig. 7c ) and was therefore allocated the largest proportion of resources. In addition, KwaZulu-Natal has a muh larger population than Mpumalanga; consequently, our results show that (given the uncertainty in province-specific pre-intervention HIV incidence estimates in women, province-specific pre-intervention HIV prevalence levels in women and province-specific levels of risk behaviour), on average, slightly more resources should be allocated to KwaZulu-Natal has a muh larger population than to Mpumalanga. In contrast, the initial optimization analysis, which did not include uncertainty, could only calculate a single GRAS. Since this was based on identifying Mpumalanga as the province where interventions would be most efficient, the GRAS was to allocate slightly more of the resources to Mpumalanga than to KwaZulu-Natal. Although our results from the multiple optimization analyses show fairly wide variation in the GRAS, our results show much lower variation in the outcome in terms of the benefit of the utilitarian plan in comparison with the egalitarian plan. Specifically, in terms of the percentage increase in HIV IP in women by the utilitarian plan in comparison with the egalitarian plan ( Table 1 ). There is less variation in the benefit because the short-term efficiency of interventions is likely to be very similar in Mpumalanga and KwaZulu-Natal ( Fig. 7a,b ); consequently, the GRAS for the utilitarian plan (over the identified range in Table 1 ) has relatively little effect on the additional number of HIV IP. If adherence is moderate the benefit of the utilitarian plan in comparison with the egalitarian plan is slightly less than when adherence is high ( Table 1 ). Notably, the results from the initial optimization analysis for the benefits of the utilitarian plan in comparison with the egalitarian plan are within the IQRs obtained from the multiple optimization analyses ( Table 1 ). Results in Fig. 9 are from the multiple optimization analyses, which include uncertainty in parameter estimation when calculating both the utilitarian and egalitarian strategy, see Methods. In both Fig. 9a,b the results for the utilitarian strategy are based on assuming that the optimal implementation plan is to divide resources between KwaZulu-Natal and Mpumalanga; the range for the GRAS that is used is shown in Table 1 . 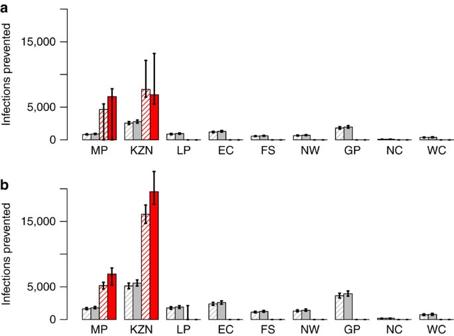Figure 9: A comparison of the number of HIV infections prevented by the utilitarian and the egalitarian strategy. The histograms in (a) show the number of HIV infections prevented in women in each province, in the first year of the rollout, assuming 50 million microbicides are available: grey data show the results of the egalitarian plan (solid grey columns based on high adherence, striped grey columns on moderate adherence) and red data show the results of the utilitarian plan (solid red columns based on high adherence, striped red columns on moderate adherence). The histograms in (b) are similar to those in (a), but are based on a supply of 100 million microbicides. In both (a) and (b) the results for the egalitarian strategy are based on the assumption that Mpumalanga and KwaZulu-Natal are the optimal two-province combination to use for geographic targeting (seeTable 1). Province abbreviations: Mpumalanga (MP), KwaZulu-Natal (KZN), Limpopo (LP), Eastern Cape (EC), Free State (FS), North West (NW), Gauteng (GP), Northern Cape (NC) and the Western Cape (WC). Figure 9a shows the number of HIV IP in women in each province in the first year of the rollout, assuming 50 million microbicides are available: grey data show the results of the egalitarian plan (solid grey columns based on high adherence, striped grey columns on moderate adherence) and red data show the results of the utilitarian plan (solid red columns based on high adherence, striped red columns on moderate adherence). The results in Fig. 9b are qualitatively similar to those shown in Fig. 9a , but they are quantitatively different as they are based on assuming 100 million microbicides are available. Clearly, HIV infections would be prevented in only two provinces if the utilitarian rollout plan is used, but in every province if the egalitarian plan were used. Not surprisingly, regardless of whether the rollout plan is based on the utilitarian or the egalitarian principle, the greater the resource constraints and/or the lower the adherence the fewer the number of HIV IP in South Africa ( Fig. 9a,b ). Figure 9: A comparison of the number of HIV infections prevented by the utilitarian and the egalitarian strategy. The histograms in ( a ) show the number of HIV infections prevented in women in each province, in the first year of the rollout, assuming 50 million microbicides are available: grey data show the results of the egalitarian plan (solid grey columns based on high adherence, striped grey columns on moderate adherence) and red data show the results of the utilitarian plan (solid red columns based on high adherence, striped red columns on moderate adherence). The histograms in ( b ) are similar to those in ( a ), but are based on a supply of 100 million microbicides. In both ( a ) and ( b ) the results for the egalitarian strategy are based on the assumption that Mpumalanga and KwaZulu-Natal are the optimal two-province combination to use for geographic targeting (see Table 1 ). Province abbreviations: Mpumalanga (MP), KwaZulu-Natal (KZN), Limpopo (LP), Eastern Cape (EC), Free State (FS), North West (NW), Gauteng (GP), Northern Cape (NC) and the Western Cape (WC). Full size image Governments in Sub-Saharan African countries may soon have to decide how best to rollout interventions to control their HIV epidemics. Our results show that the RA decisions that are made at the beginning of a rollout, and the geographic location where the rollout is initiated, will be crucial in determining the success of interventions on reducing HIV incidence rates. We have compared two different types of strategies for rolling out interventions: one (the utilitarian strategy) maximizes the number of HIV IP by using geographic targeting, and the other (the egalitarian strategy) maximizes geographic equity in access to the available resources. Notably, both of these strategies are based on ethical principles that the WHO recommends considering when deciding how to allocate scarce resources. We have found that using geographic targeting (at the level of the province) could prevent ~40% more HIV infections in the first year of the rollout than using the egalitarian plan. Our results show this would occur because there is considerable geographic variation in incidence throughout South Africa, and the efficiency of interventions increases disproportionately with increasing incidence. To increase the utility of our study, we included uncertainty in our estimates of HIV incidence rates, HIV prevalence levels and levels of risk behaviour when evaluating the potential benefits of geographic targeting (that is, the utilitarian strategy). We also included uncertainty in the rank ordering of the provinces, in terms of incidence rates. Hence we obtained probabilistic results that can be used to inform evidence-based decision-making. The purpose of our analysis was not to provide quantitative results that can be used to make detailed health policy recommendations, but to gain insights into the potential consequences of different RA strategies. Our results are robust in showing that using geographic targeting in South Africa could be an effective strategy for maximizing the impact of limited resources on controlling the HIV epidemic. Furthermore, our results indicate that microbicide-based interventions may be the most efficient in reducing HIV incidence rates in women in Mpumalanga and KwaZulu-Natal. Notably, we found that KwaZulu-Natal should receive slightly more of the resources than Mpumalanga in terms of the benefit that will be gained (in terms of the number of HIV IP) by using geographic targeting. As with any modelling study, ours has limitations. We have focused on the geographic allocation of resources when rolling out one type of intervention and not the more complex problem of how to allocate resources between different HIV prevention methods; this is the focus of our current research. We have considered only the implementation stage of the rollout; the geographic allocation of resources could be changed over subsequent years as HIV incidence rates change and/or more resources become available [10] . We have used two types of models for our analyses: a geospatial RA model coupled with a geospatial MT model. We built the geospatial RA model using parsimonious assumptions to aid the transparency of our optimization analysis. The model could be made more complex and then, in combination with optimization analyses, used to design more detailed RA strategies. These strategies could be designed to satisfy multiple objectives and/or further increase the efficiency of resource utilization by using more detailed geographic-targeting strategies; this is the focus of our current research. A more complex RA model could also be used as a foundation for detailed economic modelling [11] , [12] , [13] , [14] . Notably, the geospatial MT model that we have developed has a very different structure from previous transmission models of generalized HIV epidemics in Sub-Saharan Africa. Our novel model includes spatial demographics, geographic heterogeneity in HIV prevalence and incidence, geographic variation in treatment coverage and geographic variation in levels of risk behaviour. In contrast, previous transmission models have been built on the assumption that the population is uniformly distributed throughout the country, and the prevalence (and incidence) of HIV does not vary geographically. Notably, these assumptions do not hold for South Africa, nor for many other Sub-Saharan African countries with generalized HIV epidemics; for example, Lesotho, Botswana, Nigeria and Uganda [15] , [16] , [17] , [18] . However, we have not included several important factors such as age-structure, urban–rural differences and migration in our geospatial MT model; this would have required detailed province-specific data, which are not currently available. Increasing the complexity of our model would not change our qualitative results regarding the benefits of geographic targeting. Several strategies are being considered for controlling HIV epidemics in Sub-Saharan Africa; for example, using universal ‘test and treat’, rolling out ARV-based pre-exposure prevention tools or circumcising millions of men. It is not clear whether any of these strategies are feasible, nor whether more detailed strategies that are based on targeting ‘high-risk’ individuals [11] , [19] , [20] , [21] or discordant couples are viable [22] . The feasibility of using any type of prevention tool to control HIV epidemics will depend upon numerous factors including both acceptability and (in the case of ARV-based tools) adherence. Our results regarding geographic targeting are not specific to the rollout of interventions based on microbicides; they are generalizable to other PrEP-based prevention modalities. New drug formulations or delivery systems that do not require frequent dosing may make PrEP more acceptable, and hence overcome some of the current challenges of adherence. Recent interest has focused on the development of intra-vaginal rings for topical ARV delivery, and on novel long-acting injectable ARV formulations that provide sustained systemic drug exposures but require infrequent dosing [23] , [24] , [25] , [26] . The success of any type of public health intervention (for example, voluntary male medical circumcision, PrEP and ‘treatment as prevention’) in reducing HIV transmission will also be affected by migration, which is a fairly common phenomenon in Sub-Saharan Africa. Modelling studies have shown that migration can ‘spatially diffuse’ the impact of an intervention; that is, in the presence of migration the intervention will not be as effective in reducing transmission in the region where it is applied [27] , [28] , but could potentially reduce transmission in other regions [28] . The effect of migration on determining the success of any intervention will depend upon multiple variables: for example, the percentage of the population that are migrants, migration patterns, the length of time migrants spend away from their primary residence and the effect of migration on sexual mixing patterns. With respect to microbicides, the effect of migration will also depend on the choices women make. Some may choose to use microbicides while they are away from home, others may choose not to use them. Detailed data will need to be collected on migration to inform the design of all types of interventions in the ‘real-world’. We are the first to show that using the same amount of ARVs but different rollout plans can affect the success of interventions in controlling HIV epidemics. Specifically, we have shown that (under resource constraints) geographic targeting could be used to maximize the impact of a limited supply of resources on reducing HIV transmission. Our results indicate that further geographic targeting within provinces (that is, ‘Hot-Spots’ where incidence rates are very high) is likely to result in an even greater efficiency in resource utilization. Our qualitative findings regarding the potential utility of geographic targeting are likely to apply to other Sub-Saharan African countries that have geographic variation in the severity of their HIV epidemic; for example, Lesotho, Botswana, Nigeria and Uganda [15] , [16] , [17] , [18] . The magnitude of the difference (in terms of the number of HIV IP) between the utilitarian and egalitarian plan (that is, the benefits of using geographic targeting) will depend upon the average incidence rate in the country, the geographic variability in incidence and the level of resource constraints. The higher the overall incidence rate and/or the greater the geographic variability in incidence and/or the more constrained the resources, the more HIV infections the utilitarian rollout plan will prevent in comparison with the egalitarian plan. In contrast, the higher the treatment coverage (hence the lower the incidence), the fewer HIV infections the utilitarian rollout plan will prevent in comparison with the egalitarian plan; this is due to the nonlinear effect of incidence on efficiency. Taken together, our results have great significance for global health policy. They show that—under resource constraints—it will not be possible to maximize the efficiency of resource utilization (and hence minimize incidence) and also achieve countrywide equity in access to prevention resources. Currently, HIV prevention resources are allocated geographically with the objective of providing countrywide equity in access. However, our results suggest that many more HIV infections could be prevented—using the same amount of resources—if other ethical principles are used. Using the utilitarian principle to design rollout plans based on geographic targeting could significantly increase our ability to control HIV epidemics in Sub-Saharan Africa. Defining adherence levels and specifying effectiveness Efficacy is the degree of protection against infection conferred by a microbicide if adherence is 100%. Effectiveness is the degree of protection against infection conferred by a microbicide at a given level of adherence. The HIV effectiveness results of the CAPRISA 004 trial were reported for three adherence levels [5] . Low adherence was defined as using the microbicide in <50% of sex acts. Moderate adherence was defined as using the microbicide in 50–80% of sex acts. High adherence was defined as using the microbicide in >80% of sex acts. At low, moderate and high adherence levels the effectiveness of the microbicide in protecting against HIV infection was 28%, 38% and 54%, respectively [5] . The effectiveness of the microbicide in protecting against HSV-2 infection was 51% and was not stratified by adherence [5] . We defined three adherence levels (low, moderate and high) as in the CAPRISA trial and specified the effectiveness of the microbicide in protecting against HIV infection at each level based on the trial results [5] . On the basis of the trial results, we specified the effectiveness of the microbicide in protecting against HSV-2 infection to be 51% at all three adherence levels [5] . The geospatial MT model structure The geospatial MT model includes the spatial demographics of South Africa, the within-country geographic variation in HIV prevalence and incidence, the province-specific rollout of treatment (with coverage increasing from 2004 onwards, Supplementary Fig. 1 ) and geographic heterogeneity in sexual behaviour (see Supplementary Methods ). The model consists of 33 nonlinear ordinary differential equations. The equations specify the transmission dynamics of coupled HIV and HSV-2 epidemics; the equations are given in Section C.3.d of the Supplementary Methods . The model includes coupled HIV and HSV-2 epidemics because each virus affects the transmission of the other virus [29] , [30] , [31] , [32] . HIV infection increases the risk of transmitting HSV-2 (ref. 29 ), conversely HSV-2 infection increases the risk of transmitting HIV [33] . In addition, HSV-2 infection increases the risk of acquiring HIV [34] , [35] . All of our analyses are based on the assumption that the microbicide could potentially reduce both HIV and HSV-2 transmission; we made this assumption because the CAPRISA microbicide was found to be partially effective against both HIV and HSV-2 (ref. 5 ). The model is gender-stratified and includes susceptible individuals, individuals infected with only HIV, individuals infected with only HSV-2 and individuals co-infected with both HIV and HSV-2. The natural history of HIV is modelled as a series of three stages, characterized by CD4 level and viral load (which determines infectivity); HIV-infected individuals on treatment are also tracked. The natural history of HSV-2 is modelled as two alternating states: the infectious state (when individuals shed virus) and the noninfectious state (when the virus is latent). Individuals co-infected with both viruses are modelled to reflect modifications in infectivity and susceptibility due to HIV or HSV-2 infection. The model is based on the parsimonious assumptions that there is homogeneous mixing within a province, and negligible (at the population level) sexual mixing among individuals living in different provinces. See the Supplementary Methods for further details on model structure, a flow diagram is given in Supplementary Fig. 6 . The model was simulated using MATLAB. Model parameterization The geospatial MT model was parameterized using demographic, behavioural and treatment data from South Africa; ranges were specified for each parameter (see Section C.4 in the Supplementary Methods ). Supplementary Table 4 provides a summary of all model parameter symbols and definitions. Parameter ranges are provided in Supplementary Tables 3 and 5–7 . Province-specific parameters are provided in Supplementary Table 3 . Supplementary Table 5 gives ARV therapy and microbicide parameters. Supplementary Table 6 gives HIV parameters; Supplementary Table 7 gives HSV-2 parameters. Each parameter was sampled 1,500 times using Latin Hypercube Sampling (LHS) [36] , [37] , [38] . Model calibration and validation The parameter set, obtained using LHS [36] , [37] , [38] , was used for calibrating the geospatial MT model. Calibration was based on an iterative multi-stage procedure that includes Monte Carlo filtering; see Section C.5 in the Supplementary Methods . The model was calibrated for both women and men in each of the nine provinces for the year 2004, when HIV prevalence in South Africa appears to have stabilized ( Supplementary Fig. 7 ) and treatment was introduced. It was calibrated by fitting to gender-stratified province-specific estimates of HIV prevalence for 2004 generated by the most recent version of the Actuarial Society for South Africa (ASSA) AIDS and Demographic model [39] . The calibration resulted in 1,362 estimates for gender-stratified HIV incidence rates and prevalence levels for each of the nine provinces for the year 2004. After the model was calibrated, it was verified (see Section C.6 in the Supplementary Methods ) and validated (see Section C.7 in the Supplementary Methods ). Supplementary Figs 8 and 9 show the outputs of the calibration procedure. Multivariate sensitivity analysis We used response hypersurface modelling and LHS [36] , [37] , [38] to conduct multivariate sensitivity analyses of the geospatial MT model [36] , [40] . We determined the effect of microbicide coverage and effectiveness on reducing HIV and HSV-2 transmission in both genders over a decade in KwaZulu-Natal province. Coverage is defined as the percentage of women who are uninfected with HIV (regardless of whether they are infected with HSV-2) and who use the microbicide. We used the 1,362 simulations that had been calibrated to 2004; we introduced province-specific treatment rollout ( Supplementary Fig. 1 ), ran the simulations to the current year and then introduced microbicide-based interventions. The parameter values used are specific to KwaZulu-Natal; see Supplementary Table 3 . The rollout of microbicides was modelled for 10 years; see Section C.2 in Supplementary Methods and Supplementary Fig. 8 . Throughout this time we also modelled the planned continued expansion of treatment; see Section C.1 in the Supplementary Methods and Supplementary Fig. 1 . We varied microbicide coverage rates from 30 to 90%, HIV effectiveness from 15 to 75% and HSV-2 effectiveness from 30 to 75%. The reduction in HIV and HSV-2 transmission due to microbicides, over a decade, was calculated. Response hypersurfaces were then fitted to these results. Scenario analyses We conducted scenario analyses of the geospatial MT model to examine the effect of microbicide coverage and effectiveness on reducing HIV and HSV-2 transmission in KwaZulu-Natal province where the CAPRISA 004 trial was conducted. The six scenarios are based on different assumptions regarding coverage (60 or 90%) and adherence (low, moderate or high). Low, moderate and high adherence corresponds to an effectiveness of the microbicide in protecting against HIV infection of 28%, 38% and 54%, respectively. In all six scenarios, the effectiveness of the microbicide in protecting against HSV-2 infection is 51%. The remaining parameter values used to generate the scenarios are the median values of the distributions shown in Supplementary Tables 3 and 5–7 . Uncertainty analyses We conducted four uncertainty analyses of the geospatial MT model. These analyses were based on: (i) high coverage (90%) and high adherence, (ii) high coverage (90%) and moderate adherence, (iii) moderate coverage (60%) and high adherence and (iv) moderate coverage (60%) and moderate adherence. The adherence–effectiveness relationship we modelled was determined from the results of the CAPRISA trial [5] . To model high adherence, we used a triangular distribution for effectiveness against HIV ranging from 34 to 74% with a peak density at 54% (ref. 5 ). To model moderate adherence, we used a triangular distribution for effectiveness against HIV ranging from 18 to 58% with a peak density at 38% [5] . For all four uncertainty analyses, we used a triangular distribution for effectiveness against HSV-2 ranging from 31 to 71% with a peak density at 51% (ref. 5 ). For each uncertainty analysis, and for each of the nine provinces, we used the 1,362 simulations that had been obtained from the calibration procedure. The model had been calibrated to 2004 when the rollout of treatment began in South Africa. Therefore, we introduced treatment into each of the simulations beginning in 2004. We used different treatment rollout rates in each province; see Section C.1 of the Supplementary Methods and Supplementary Fig. 1 . We continued modelling the rollout of treatment in each province to the current year at which point we introduced interventions. Therefore we had 1,362 estimates for the gender-stratified pre-intervention HIV incidence rates and prevalence levels in each province. The GRAS for the egalitarian rollout plan was used to divide the available supply of microbicides among the nine provinces. The proportion of the supply that each province was allocated equaled the number of HIV-negative women who live in the province divided by the total number of HIV-negative women who live in SA. The modelling of the rollout of microbicides is described in Section C.2 of the Supplementary Methods , and shown in Supplementary Fig. 10 . When conducting the uncertainty analyses, as well as the historical rollout of treatment beginning in 2004, we included the planned province-specific expansion of treatment; see Section C.1 of the Supplementary Methods and Supplementary Fig. 1 . Predictive maps of the cumulative number of HIV IP We used the uncertainty analyses to predict the cumulative number of HIV IP (over a decade) by interventions in each province. When we made predictions we excluded the effect of expanding treatment coverage on reducing transmission. This was accomplished by running each scenario in each uncertainty analysis twice: once with interventions and expanding treatment coverage, and once with only expanding treatment coverage. The difference between the two scenarios is the number of HIV IP by microbicide-based interventions. Results from these analyses were then mapped. Intervention efficiency maps Predictions generated by the uncertainty analyses were used to calculate the long-term (that is, over a decade) efficiency of interventions in reducing HIV transmission in both genders in each province; the results were then mapped. Long-term efficiency was defined as the number of women-years on microbicide needed to prevent one HIV infection in either gender. Women-years were calculated by multiplying the number of women using microbicides each year with the number of years of microbicide usage. Pre-intervention incidence rate and long-term efficiency Predictions generated by the uncertainty analyses were plotted and used to identify a statistical relationship between the pre-intervention HIV incidence rate and the long-term efficiency of interventions in reducing HIV transmission in both genders. We also conducted regression analyses to determine the value of y : where y represents the median number of women-years necessary to prevent one HIV infection in women. We determined the value of y assuming either high or moderate adherence. On the basis of the data from the CAPRISA trial [5] , we assume high adherence corresponds to using microbicides in 85% of sex acts and moderate adherence to using microbicides in 65% of sex acts. Short-term efficiency of interventions The predictions generated by the uncertainty analyses were used to calculate the short-term efficiency of interventions (that is, the efficiency in the first year of the rollout) in each province. Short-term efficiency was defined as the number of HIV IP per 10,000 microbicides used. This equals 10,000/2y cau where y represents the median number of women-years necessary to prevent one HIV infection in women and 2cau is the total number of microbicides used (on average) per year by each woman. In the expression 2cau , c is the average number of new sex partners per woman per year, a the number of sex acts per partnership and u the proportion of sex acts for which microbicides are used according to the CAPRISA 004 protocol (hence, u represents adherence). Since the protocol was based on using a microbicide before and after sex [5] , the factor 2 is included in the equation. We calculated the short-term efficiency of interventions in each province by using province-specific values for y and c . We calculated province-specific estimates of y by dividing the number of HIV IP by the number of women-years on microbicide for each of the 1,362 simulations. Province-specific values for c were estimated during the calibration of the geospatial MT model; the range is given in Supplementary Table 3 . The range of estimates for a is given in Supplementary Table 6 . We calculated short-term efficiency of interventions assuming either high or moderate adherence. On the basis of data from the CAPRISA trial [5] , we assume high adherence corresponds to using microbicides in 85% of sex acts and moderate adherence to using microbicides in 65% of sex acts. Structure of the geospatial RA model The geospatial RA model was based on the parsimonious assumption that, over 1 year, HIV prevalence does not change substantially and the number of HIV IP in men (due to women using microbicides) would be negligible. The model operates under two constraints: the total number of microbicides that are available in the first year of the rollout (that is, the amount of resources) and adherence. Model parameterization The geospatial RA model was parameterized using province-specific estimates for the number of 15–49-year-old HIV-negative women residing in the province, the average number of new sex partners per woman per year and the pre-intervention HIV incidence rate in women. The number of 15–49-year-old HIV-negative women in each province was calculated by multiplying the total number of 15–49-year-old women in the province with the proportion of women in that province that are not infected (that is, one minus the pre-intervention HIV prevalence level). The total number of 15–49-year-old women in each province was based on estimates from the most recent version of the ASSA AIDS and Demographic model [39] . Ranges for province-specific estimates for the average number of new sex partners per woman per year were obtained from the calibration of the geospatial MT model. Pre-intervention HIV incidence rates and prevalence levels were obtained from the uncertainty analyses of the geospatial MT model. Estimating the GRAS for the egalitarian rollout plan Under the egalitarian rollout plan the supply of resources (that is, microbicides) is divided among the nine provinces in proportion to the number of women in need of protecting against HIV infection. Specifically, the percentage of the supply that a province is allocated is equal to the number of 15–49-year-old HIV-negative women who live in that province divided by the total number of HIV-negative women (in the same age group) who live in SA. For each province, we calculated the number of HIV-negative women in the province by multiplying the number of 15–49-year-old women in the province [39] with the proportion of women in that province that are not infected (that is, one minus the pre-intervention HIV prevalence level). The total number of 15–49-year-old women in each province was based on estimates generated by the most recent version of the ASSA AIDS and Demographic model [39] . We calculated a GRAS for the egalitarian plan that included uncertainty in estimating the pre-intervention HIV prevalence levels in women, and another without uncertainty. To include uncertainty, we used province-specific ranges for the pre-intervention HIV prevalence levels obtained from the uncertainty analyses of the geospatial MT model. To calculate the GRAS for the egalitarian plan without uncertainty we used the median value of the range for each province. Calculating the number of HIV IP by the egalitarian plan The number of HIV IP in each of the nine provinces (under the egalitarian plan) is calculated as the product of the number of HIV-negative women (aged 15–49 years) who reside in that province, the pre-intervention incidence rate in that province, the proportion of HIV-negative women (in that province) who use microbicides and the effectiveness of the microbicide. Summing over all provinces gives the total number of HIV IP. Optimization without uncertainty in parameter estimation Throughout our description of the optimization analyses when we refer to women, we are referring to women who are 15–49 years old. We used the geospatial RA model and mathematical optimization techniques based on linear programming to calculate (under resource constraints) the GRAS that is necessary to implement the utilitarian rollout plan, the optimal geographic location to initiate a rollout based on the utilitarian principle and the number of HIV IP in women in the first year of the rollout. We used the total number of HIV IP in women in South Africa as the objective function for the optimization analysis, and specified the resource constraint in terms of the total number of microbicides available in the first year of the rollout. The optimal solution is the GRAS that maximizes the total number of HIV IP in South Africa in the first year of the rollout; that is, it is the GRAS for the utilitarian rollout plan. As the geospatial RA model considers only the first year of the rollout, the province(s) that are allocated resources in the optimal solution are the optimal geographic location(s) to initiate the rollout. The optimization algorithm allocates the available resources disproportionally to the provinces where interventions are the most efficient; that is, to the provinces that prevent the highest number of HIV infections for a given amount of resources. The efficiency of interventions in a province is equal to the number of HIV IP in that province in the first year of the rollout divided by the total number of microbicides used in that province. The number of HIV IP in each province, given a specific proportion of the supply of microbicides, is calculated as the product of the number of HIV-negative women who reside in the province, the HIV incidence rate in the absence of microbicides, the proportion of HIV-negative women who use microbicides and the level of adherence (which specifies the degree of effectiveness of the microbicide in protecting against HIV). The total number of microbicides used in each province is calculated as the product of the number of HIV-negative women who reside in that province, the proportion of these women who use microbicides, the average number of new sex partners per woman per year and twice the average number of sex acts per partnership. We assume women will use microbicides according to the CAPRISA 004 protocol (that is, once before and after sex [5] ). The optimization algorithm identifies the GRAS that would maximize the number of HIV IP in SA in the first year of a rollout. The optimization problem can be stated as the following linear program: where N i =number of women who reside in the i th province, P i =HIV prevalence in women in the i th province at the beginning of the rollout, I i =pre-intervention HIV incidence rate in women in the i th province, p =effectiveness of the microbicide in protecting against HIV infection, x i =proportion of eligible women in the i th province that receive microbicides in the first year of the rollout, c i =average number of new sex partners per woman per year in the i th province, a =average number of sex acts per partnership for women, u =adherence level, Y =total number of microbicides available in SA in the first year of the rollout (that is, resource constraint). For each of the nine provinces, we used the parameter set (out of the 1,362 parameter sets obtained from calibrating the model) that generated the median value for the incidence rate. With these nine parameter sets, we used the geospatial MT model to calculate—for each province—the number of 15–49-year-old women living in that province at the beginning of the rollout, the pre-intervention HIV prevalence level in women, the pre-intervention HIV incidence rate in women and the average annual number of new sex partners ( N i ,P i ,I i and c i for i =1..9, respectively). The x term is the result of the optimization, it specifies the proportion of eligible women in each province that receive microbicides in the first year of the rollout to maximize the total number of HIV IP in SA in the first year of the rollout. Hence it specifies the GRAS for the utilitarian rollout plan. We calculated the GRAS under two levels of resource constraints, assuming either 50 or 100 million microbicides were available. Fifty million is enough for ~33%, and 100 million for ~66% of the 15–49-year-old HIV-negative women in SA. For each level of resource constraint we conducted two analyses, assuming either high or moderate adherence. On the basis of the data from the CAPRISA trial [5] , we assume high adherence corresponds to using microbicides in 85% of sex acts (resulting in an effectiveness against HIV infection of 54%) and moderate adherence to using microbicides in 65% of sex acts (resulting in an effectiveness against HIV infection of 38%). Optimization including uncertainty in parameter estimation We also conducted multiple (1,362) optimization analyses that included uncertainty in estimating the values of the province-specific pre-intervention HIV incidence rates in women, the pre-intervention HIV prevalence levels in women and the average number of new sex partners per woman per year. We also included uncertainty in the number of sex acts per partnership. We included uncertainty by using parameter ranges. We used province-specific ranges for the pre-intervention HIV incidence rates and prevalence levels obtained from the uncertainty analyses of the geospatial MT model. Province-specific ranges for the average number of new sex partners per woman per year are given in Supplementary Table 3 . The range for the average number of sex acts per partnership is given in Supplementary Table 6 . In each of the optimization analyses the rank ordering of the provinces, in terms of incidence rates in women, was varied probabilistically. How to cite this article : Gerberry, D. J. et al. Using geospatial modelling to optimize the rollout of antiretroviral-based pre-exposure HIV interventions in Sub-Saharan Africa. Nat. Commun. 5:5454 doi: 10.1038/ncomms6454 (2014).